The orphan receptor Gpr83 regulates systemic energy metabolism via ghrelin-dependent and ghrelin-independent mechanisms The G protein-coupled receptor 83 (Gpr83) is widely expressed in brain regions regulating energy metabolism. Here we report that hypothalamic expression of Gpr83 is regulated in response to nutrient availability and is decreased in obese mice compared with lean mice. In the arcuate nucleus, Gpr83 colocalizes with the ghrelin receptor (Ghsr1a) and the agouti-related protein. In vitro analyses show heterodimerization of Gpr83 with Ghsr1a diminishes activation of Ghsr1a by acyl-ghrelin. The orexigenic and adipogenic effect of ghrelin is accordingly potentiated in Gpr83 -deficient mice. Interestingly, Gpr83 knock-out mice have normal body weight and glucose tolerance when fed a regular chow diet, but are protected from obesity and glucose intolerance when challenged with a high-fat diet, despite hyperphagia and increased hypothalamic expression of agouti-related protein, Npy, Hcrt and Ghsr1a. Together, our data suggest that Gpr83 modulates ghrelin action but also indicate that Gpr83 regulates systemic metabolism through other ghrelin-independent pathways. The murine G protein-coupled receptor (GPCR) 83 (Gpr83) is an orphan receptor belonging to the rhodopsin-like or family A of GPCRs [1] . This family is by far the largest subfamily of GPCRs and includes several receptors implicated in the regulation of systemic metabolism, such as the ghrelin receptor (Ghsr1a) [2] , [3] and the orexin receptors 1 and 2 (Ox1r and Ox2r) [4] . Gpr83 was originally identified as a glucocorticoid-induced transcript in a murine T cell line and, therefore, was referred to as glucocorticoid-induced receptor [5] . Induction of Gpr83 mRNA expression following dexamethasone [6] or amphetamine [7] treatment suggests a possible role in the regulation of the hypothalamus–pituitary–adrenal axis. This possibility is further supported by the observation that Gpr83 is expressed in hypothalamic nuclei that govern energy balance, such as the arcuate nucleus (ARC), the paraventricular nucleus and the lateral hypothalamic area [6] , [8] , [9] , [10] . As Gpr83 is expressed in hypothalamic nuclei relevant for energy metabolism control and as a potential modulator of the hypothalamus–pituitary–adrenal axis might also be relevant for systems metabolism, we hypothesized that Gpr83 might have a role in the central regulation of energy metabolism. To test this hypothesis, we analysed the expression of Gpr83 in the mouse hypothalamus and observed that its expression is regulated by nutrient availability. In the ARC, we further find Gpr83 being colocalized with both the ghrelin receptor (Ghsr1a) and the agouti-related protein (AgRP), and in vitro analysis in HEK293 and mouse hypothalamic N41 cells show heterodimerization of Gpr83 with Ghsr1a that reduces ghrelin receptor activity. In line with this observation, the effects of ghrelin treatment on food intake and adiposity are enhanced in Gpr83 knock-out (Gpr83 ko) mice, thus supporting a functional interaction between Gpr83 and Ghsr1a in vivo . However, Gpr83 ko mice are also protected from obesity and glucose intolerance following exposure to high-fat diet (HFD), despite relative hyperphagia and increased hypothalamic expression of AgRP, Npy, Hcrt and Ghsr1a. Taken together, these data suggest that Gpr83 has multiple ghrelin-dependent and ghrelin-independent roles in the regulation of systemic energy metabolism. Colocalization of Gpr83 with Ghsr1a and AgRP Gene expression profiling in C57BL/6 mice confirmed that Gpr83 is predominantly expressed in the brain, with moderate expression in the hypothalamus. In line with previous studies [7] , no expression was observed in peripheral tissues, such as the liver, muscle, heart, testis, as well as the white and brown adipose tissue ( Fig. 1a ). Of appreciable note, analysis of hypothalamic Gpr83 expression revealed a decrease in mice with diet-induced obesity as compared with age-matched, lean controls ( Fig. 1b ). Furthermore, fasting of lean mice for 12, 24 or 36 h resulted in a time-dependent decrease in the hypothalamic expression of Gpr83 ( Fig. 1c ). Refeeding with either a HFD or a fat-free diet for 6 h caused a subsequent increase in hypothalamic Gpr83 mRNA expression ( Fig. 1c ). In situ hybridization histochemistry in combination with immunohistochemistry revealed a broad abundance of Gpr83 in the ARC. In particular, we found Gpr83 expressed in specific subsets of ARC neurons that express Ghsr1a ( Fig. 2a–c ) and AgRP ( Fig. 2d ). 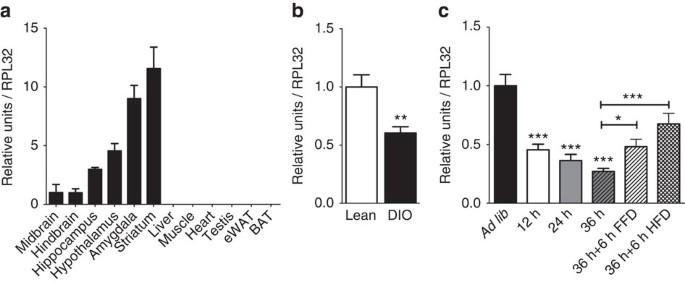Figure 1: Gene expression profiling of Gpr83 in C57BL/6 mice. Expression pattern of Gpr83 in different brain areas, as well as in peripheral tissues (a). Hypothalamic expression of Gpr83 in diet-induced obese (DIO) compared with lean mice (N=6–8 mice per group) (b). Hypothalamic expression of Gpr83 in response to fasting for 12, 24 or 36 h, and after refeeding for 6 h with either a high-fat diet (HFD) or a fat-free diet (FFD,N=6–8 mice per group) (c). *P<0.05, **P<0.01, ***P<0.001 based on unpaired two-tailed Student’st-test (b) or one-way analysis of variance followed by Newman-Keuls multiple comparison test (c). Data represent means±s.e.m.Ab lib,ad libitum. Figure 1: Gene expression profiling of Gpr83 in C57BL/6 mice. Expression pattern of Gpr83 in different brain areas, as well as in peripheral tissues ( a ). Hypothalamic expression of Gpr83 in diet-induced obese (DIO) compared with lean mice ( N =6–8 mice per group) ( b ). Hypothalamic expression of Gpr83 in response to fasting for 12, 24 or 36 h, and after refeeding for 6 h with either a high-fat diet (HFD) or a fat-free diet (FFD, N =6–8 mice per group) ( c ). * P <0.05, ** P <0.01, *** P <0.001 based on unpaired two-tailed Student’s t -test ( b ) or one-way analysis of variance followed by Newman-Keuls multiple comparison test ( c ). Data represent means±s.e.m. Ab lib , ad libitum. 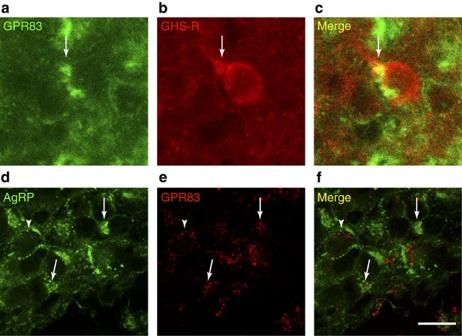Figure 2: Gpr83 abundance in the arcuate nucleus of the hypothalamus. Dual labelling byin situhybridization histochemistry for Gpr83 and immunohistochemistry for Ghsr and AgRP. Gpr83 locates in ghrelin receptor expressing neurons (a–c) or AgRP neurons (d–f) in the arcuate nucleus of the hypothalamus. Scale bar, 20 μm in (a–c) and 50 μm in (d–f). Full size image Figure 2: Gpr83 abundance in the arcuate nucleus of the hypothalamus. Dual labelling by in situ hybridization histochemistry for Gpr83 and immunohistochemistry for Ghsr and AgRP. Gpr83 locates in ghrelin receptor expressing neurons ( a – c ) or AgRP neurons ( d – f ) in the arcuate nucleus of the hypothalamus. Scale bar, 20 μm in ( a – c ) and 50 μm in ( d – f ). Full size image Heterodimerization of Gpr83 and Ghsr1a To determine whether Gpr83 influences ghrelin–Ghsr1a signalling, we next examined whether both receptors interact in vitro . Both sandwich enzyme-linked immunosorbent assay (ELISA) and a yellow fluorescent protein (YFP)-based protein complementation assay (YFP-PCA) revealed heterodimerization of Gpr83 and Ghsr1a ( Fig. 3a ). Furthermore, cotransfection of Ghsr1a and Gpr83 in HEK293 cells led to a 43% reduction in ghrelin-stimulated Ghsr1a activity compared with control cells cotransfected with Ghsr1a and the rat muscarinic acetylcholine receptor M 3 (rM3R) ( Fig. 3c ). Of appreciable note, this effect was not due to changes in the cell surface or total Ghsr1a expression ( Fig. 3d ), and Gpr83 activity was not influenced by treatment with acyl ghrelin, des-acyl ghrelin or obestatin ( Supplementary Fig. S1A ). Furthermore, heterodimerization of Gpr83 and Ghsr1a was also observed in mouse hypothalamic N41 cells cotransfected with Ghsr1a and Gpr83 ( Supplementary Fig. S1B ). Together, these data indicate that Gpr83–Ghsr1a heterodimerization reduces activation of Ghsr1a by ghrelin, thus supporting a possible role for Gpr83 in the regulation of energy homeostasis by reducing the ability of ghrelin to activate its only known endogenous receptor. 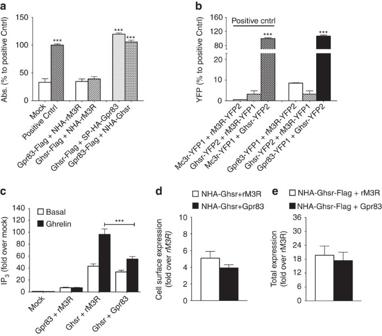Figure 3: mGpr83 forms heterodimers with mGhsr and modifies its signalling properties. Cells were transiently cotransfected with equal amounts of differentially taggedGpr83andGhsr, respectively.Sandwich ELISA studies in COS-7 cells, expressed as % absorption (492 nm/620 nm) relative to positive control (NHA-Mc3r+Ghsr-Flag) and mock (NHA-Ghsr) (a). YFP-based protein complementation assay in HEK293 cells, expressed as % fluorescent cells to positive control (Mc3r-YFP1+Ghsr-YFP2) (b) and functional characterization of the Ghsr/Gpr83 heterodimer in HEK293 (c). Measurement of inositol-3 phosphate (IP3) following stimulation with 1,000 nM ghrelin was carried out 48 h after transfection. (d) HA-tags of receptors on the cell surface in comparison with untagged rM3R as negative control. (e) HA- and Flag-double tagged receptors expressed as fold over the rM3R negative control (e,d). Data were assessed from a minimum of three independent experiments (a–e), each performed at least in triplicates (a,c–e). Cntrl, control; rM3R, rat muscarinic acetylcholine receptor M3. Data represent mean±s.e.m. ***P<0.001 based on one-way analysis of variance followed by Bonferroni’spost-hoctest. Figure 3: mGpr83 forms heterodimers with mGhsr and modifies its signalling properties. Cells were transiently cotransfected with equal amounts of differentially tagged Gpr83 and Ghsr , respectively. S andwich ELISA studies in COS-7 cells, expressed as % absorption (492 nm/620 nm) relative to positive control (NHA-Mc3r+Ghsr-Flag) and mock (NHA-Ghsr) ( a ). YFP-based protein complementation assay in HEK293 cells, expressed as % fluorescent cells to positive control (Mc3r-YFP1+Ghsr-YFP2) ( b ) and functional characterization of the Ghsr/Gpr83 heterodimer in HEK293 ( c ). Measurement of inositol-3 phosphate (IP 3 ) following stimulation with 1,000 nM ghrelin was carried out 48 h after transfection. ( d ) HA-tags of receptors on the cell surface in comparison with untagged rM3R as negative control. ( e ) HA- and Flag-double tagged receptors expressed as fold over the rM3R negative control ( e , d ). Data were assessed from a minimum of three independent experiments ( a – e ), each performed at least in triplicates ( a , c – e ). Cntrl, control; rM3R, rat muscarinic acetylcholine receptor M 3 . Data represent mean±s.e.m. *** P <0.001 based on one-way analysis of variance followed by Bonferroni’s post-hoc test. Full size image Metabolic phenotype of chow-fed Gpr83 ko mice To determine whether Gpr83 has a role in regulating systemic metabolism in vivo , we next assessed the metabolic phenotype of Gpr83-deficient (Gpr83 ko) mice. These mice had normal body weight, food intake, glucose tolerance and insulin sensitivity when fed a regular chow diet ( Fig. 4 ), whereas free-fatty acids (FFA) were increased under the same conditions ( Table 1 ). Compared with wild-type (wt) control mice, body fat mass ( Fig. 4b ) and plasma leptin levels ( Table 1 ) were moderately decreased without any notable difference in lean tissue mass ( Fig. 4c ). These data suggest that under normal feeding conditions, Gpr83 may be involved in regulating lipolysis. No difference between chow-fed mice was observed in basal plasma levels of insulin, insulin-like growth factor 1, growth hormone (GH), cholesterol or triglycerides ( Table 1 ). 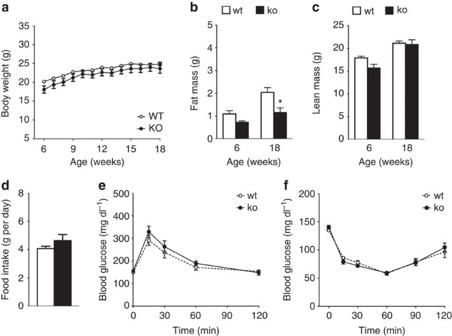Figure 4: Metabolic phenotype of chow-fed global Gpr83 ko mice. Body weight (a), body composition (b,c), food intake (d), as well as glucose tolerance (ipGTT, 1.5 g glucose per g body weight) (e) and insulin sensitivity (ipITT) (f) of Gpr83 ko (N=7) and wt (N=9) mice fed with a regular chow diet. *P<0.05 based on unpaired two-sided Student’st-test. Data represent means±s.e.m. Figure 4: Metabolic phenotype of chow-fed global Gpr83 ko mice. Body weight ( a ), body composition ( b , c ), food intake ( d ), as well as glucose tolerance (ipGTT, 1.5 g glucose per g body weight) ( e ) and insulin sensitivity (ipITT) ( f ) of Gpr83 ko ( N =7) and wt ( N =9) mice fed with a regular chow diet. * P <0.05 based on unpaired two-sided Student’s t -test. Data represent means±s.e.m. Full size image Table 1 Plasma analysis of chow-fed Gpr83 ko and wt mice treated chronically icv with either ghrelin or saline. Full size table Acute and chronic ghrelin treatment in Gpr83 ko mice To test the hypothesis that Gpr83 deficiency in adult mice would enhance ghrelin action through uninhibited ghrelin-receptor signalling, we measured acute food intake in chow-fed Gpr83 ko and wt mice following a single intraperitoneal injection of ghrelin (4.8 μmol kg −1 ) or saline. Following ghrelin treatment, acute food intake was significantly higher in Gpr83 ko mice compared with that of wt controls ( Fig. 5a ), although there was a similar response in ghrelin-induced GH secretion ( Fig. 5b ). Of appreciable note, twice-daily subcutaneous ghrelin treatment (2.4 μmol kg −1 per day) of HFD fed Gpr83 ko and wt mice for 6 days revealed a greater increase in food intake in the Gpr83 ko mice ( Fig. 5c ). 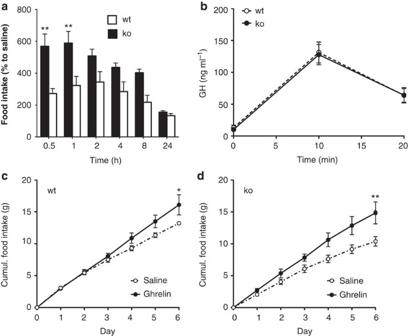Figure 5: Food intake after peripheral ghrelin treatment in Gpr83 ko mice. Acute food intake (% to saline treated mice) of chow-fed Gpr83 ko and wt mice treated with a single intraperitoneal (i.p.) injection of ghrelin (4.8 μmol kg−1) or saline (N=5–7 mice per group) (a). Ghrelin induced GH secretion of chow-fed Gpr83 ko and wt mice following single i.p. treatment with ghrelin (4.8 μmol kg−1,N=8–17 mice per group) (b). Cumulative food intake of HFD-fed Gpr83 ko and wt mice treated for 6 days via twice daily subcutaneous injection of either ghrelin (2.4 μmol kg−1per day) or saline (N=4–8 mice per group) (c,d). Data represent mean±s.e.m. *P<0.05, **P<0.01 based on two-way analysis of variance followed by Bonferronipost-hoctest. Figure 5: Food intake after peripheral ghrelin treatment in Gpr83 ko mice. Acute food intake (% to saline treated mice) of chow-fed Gpr83 ko and wt mice treated with a single intraperitoneal (i.p.) injection of ghrelin (4.8 μmol kg −1 ) or saline ( N =5–7 mice per group) ( a ). Ghrelin induced GH secretion of chow-fed Gpr83 ko and wt mice following single i.p. treatment with ghrelin (4.8 μmol kg −1 , N =8–17 mice per group) ( b ). Cumulative food intake of HFD-fed Gpr83 ko and wt mice treated for 6 days via twice daily subcutaneous injection of either ghrelin (2.4 μmol kg −1 per day) or saline ( N =4–8 mice per group) ( c , d ). Data represent mean±s.e.m. * P <0.05, ** P <0.01 based on two-way analysis of variance followed by Bonferroni post-hoc test. Full size image As the effects of ghrelin on appetite and energy homeostasis are mediated by the central nervous system, we next implanted osmotic minipumps to allow chronic intracerebroventricular (icv) infusion of ghrelin (5 nmol per day) into chow-fed Gpr83 ko mice and matched wt controls. Under these conditions, ghrelin treatment led to a greater increase in body weight ( Fig. 6a ), food intake ( Fig. 6c ) and fat mass ( Fig. 6e ) in Gpr83 ko mice as compared with that of wt controls. Consistent with the greater increase in fat mass following ghrelin treatment, plasma leptin was also increased significantly in Gpr83 ko but not in wt mice, whereas FFA levels were decreased ( Table 1 ). Taken together, these data suggest that Gpr83 expression in the central nervous system reduces the response to ghrelin in vivo . 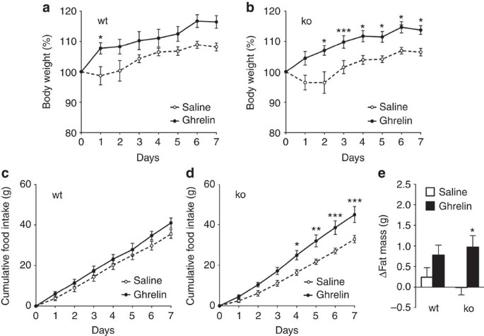Figure 6: Effects of central ghrelin treatment in Gpr83 ko mice. Body weight (a,b), cumulative food intake (c,d) and change of fat mass (e) of Gpr83 ko and wt mice treated chronically for 7 days via icv ghrelin infusion (5 nmol per day) in the lateral ventricle (N=6–7 mice per group). *P<0.05; **P<0.01; ***P<0.001 based on 2-way ANOVA followed by Bonferronipost-hoctest (a–d) or unpaired 2-tailed Student’st-test (e). 2-way ANOVA p-value for overall treatment isP=0.027 (a),P=0.0047 (b),P=0.241 (c) andP=0.0082 (d). Data represent mean±s.e.m. Figure 6: Effects of central ghrelin treatment in Gpr83 ko mice. Body weight ( a , b ), cumulative food intake ( c , d ) and change of fat mass ( e ) of Gpr83 ko and wt mice treated chronically for 7 days via icv ghrelin infusion (5 nmol per day) in the lateral ventricle ( N =6–7 mice per group). * P <0.05; ** P <0.01; *** P <0.001 based on 2-way ANOVA followed by Bonferroni post-hoc test ( a – d ) or unpaired 2-tailed Student’s t -test ( e ). 2-way ANOVA p-value for overall treatment is P =0.027 ( a ), P =0.0047 ( b ), P =0.241 ( c ) and P =0.0082 ( d ). Data represent mean±s.e.m. Full size image Gpr83 ko mice are protected from diet-induced obesity As both body fat mass and plasma leptin levels were decreased in chow-fed Gpr83 ko mice, we investigated whether loss of Gpr83 protects against the effects of chronic HFD exposure. Indeed, after 18 weeks of HFD exposure, body weight remained significantly decreased in Gpr83 ko mice compared with wt controls ( Fig. 7a ). This decreased body weight was reflected in decreased body fat, but not in lean tissue mass ( Fig. 7b ). Gpr83 ko mice further showed an improved glucose tolerance ( Fig. 7d ) without a change in insulin sensitivity ( Fig. 7e ). Surprisingly, however, food intake was increased in the Gpr83 ko mice compared with that in wt controls ( Fig. 7f–g ). Consistent with this effect, expression of AgRP, Npy, Hcrt and Ghsr1a were increased in the hypothalamus of the Gpr83 ko mice ( Fig. 7h ), notably, without any difference in plasma levels of des-acyl or acyl ghrelin ( Fig. 7i ). Measurement of energy metabolism followed by analysis of covariance analysis (as previously suggested [11] ) further revealed that energy expenditure is increased in HFD-fed Gpr83 ko mice ( Fig. 7j ), notably, without changes in locomotor activity ( Fig. 7l ). No overall difference was further observed in the respiratory quotient (RQ), despite significantly increased RQ during the dark phase ( Fig. 7m ). Taken together, these data indicate that in addition to modulating ghrelin action, Gpr83 influences systemic energy metabolism, particularly in response to HFD exposure. 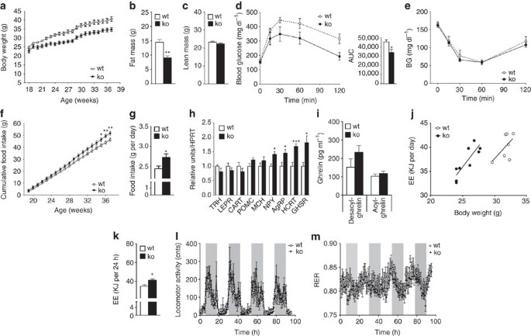Figure 7: Metabolic phenotype of global Gpr83 ko mice after HFD exposure. Body weight (a), body composition (b,c), glucose tolerance (ipGTT, 1.5 g glucose per g body weight) (d), insulin sensitivity (ipITT) (e), as well as food intake (f,g) of Gpr83 ko and wt mice fed with a HFD. Hypothalamic expression pattern of genes related to food intake (h) plasma levels of acyl- and desacyl ghrelin (i), as well as measurement of energy expenditure (j,k), locomotor activity (l) and RQ (m) in Gpr83 ko and matched wt control mice fed with a HFD. Panels (a–h) and (j–m) and containN=5–9 mice each genotype, PanelicontainsN=7–16 mice each genotype. Data in panel (h) are normalized to housekeeping gene hypoxanthine phosphoribosyltransferase 1 (HPRT). *P<0.05, **P<0.01, ***P<0.001 based on unpaired two-tailed Student’st-test (b,d,g,h,k) or two-way analysis of variance followed by Bonferronipost-hoctest (f). Data represent means±s.e.m. Figure 7: Metabolic phenotype of global Gpr83 ko mice after HFD exposure. Body weight ( a ), body composition ( b , c ), glucose tolerance (ipGTT, 1.5 g glucose per g body weight) ( d ), insulin sensitivity (ipITT) ( e ), as well as food intake ( f , g ) of Gpr83 ko and wt mice fed with a HFD. Hypothalamic expression pattern of genes related to food intake ( h ) plasma levels of acyl- and desacyl ghrelin ( i ), as well as measurement of energy expenditure ( j , k ), locomotor activity ( l ) and RQ ( m ) in Gpr83 ko and matched wt control mice fed with a HFD. Panels ( a – h ) and ( j – m ) and contain N =5–9 mice each genotype, Panel i contains N =7–16 mice each genotype. Data in panel ( h ) are normalized to housekeeping gene hypoxanthine phosphoribosyltransferase 1 (HPRT). * P <0.05, ** P <0.01, *** P <0.001 based on unpaired two-tailed Student’s t -test ( b , d , g , h , k ) or two-way analysis of variance followed by Bonferroni post-hoc test ( f ). Data represent means±s.e.m. Full size image Heterodimerization of Gpr83 with Mc3r As our data point to a more complex role of Gpr83 in systems metabolism, we next tested the hypothesis that Gpr83 might also interact with other hypothalamic GPCRs. Accordingly, based on previous reports indicating that Ghsr1a interacts with the melanocortin 3 receptor (Mc3r) [12] , we next analyzed heterodimer formation between Gpr83 and Mc3r in vitro . Both sandwich ELISA and YFP-PCA revealed a robust interaction between Gpr83 and Mc3r ( Supplementary Fig. S2A,B ). Furthermore, α-melanocyte-stimulating hormone stimulation of COS-7 cells cotransfected with Gpr83 and Mc3r led to a two-fold increase in cAMP accumulation compared with cells transfected with Mc3r alone ( Supplementary Fig. S2C ). The same results were observed after stimulation with the selective Mc3r ligand γ-melanocyte-stimulating hormone (data not shown). Again, these effects were not due to changes in cell surface or total expression of Mc3r ( Supplementary Fig. S2D,E ). These data are consistent with a more complex role for Gpr83 in the regulation of energy metabolism and point to its interaction with multiple other relevant receptors. Previous studies have shown that Gpr83 is widely distributed in the brain, including hypothalamic nuclei governing energy balance, thus suggesting a role of Gpr83 in the neuroendocrine control of energy metabolism. Here we show for the first time that in the ARC, Gpr83 is colocalized with the ghrelin receptor (Ghsr1a) and AgRP, and that hypothalamic expression of Gpr83 is tightly regulated in response to fasting and refeeding. In vitro analysis further revealed that Gpr83 forms heterodimer with Ghsr1a and that concomitant overexpression of both receptors led to an inhibition of the acyl-ghrelin-mediated activation of Ghsr1a, both in HEK293 cells and in mouse hypothalamic N41 cells. Together, these data indicate that the Gpr83/Ghsr1a dimerization affects ghrelin’s ability to activate its only known endogenous receptor. The functional interaction of Gpr83 and Ghsr1a is further supported by in vivo analysis showing a superior effect of ghrelin treatment on body weight, body fat mass and food intake in Gpr83 ko compared with that of wt mice. However, although our data strongly indicate a functional interaction of Gpr83 and Ghsr1a, further analyses are warranted to narrow down the molecular pathways of Gpr83 signalling. The decreased body fat mass with decreased plasma concentrations of leptin and increased levels FFAs observed here in the Gpr83 ko mice indicate that Gpr83 is also implicated in lipid utilization. The observation of increased food intake and expression of AgRP, Npy, Hcrt and Ghsr1a in HFD-fed Gpr83 ko mice is consistent with our in vitro and in vivo data, indicating that ghrelin signalling is increased in these ko animals and suggests an important role of GPCR dimerization for body weight maintenance. However, the observed increase in energy metabolism when Gpr83 ko mice are fed an HFD suggests that additional Gpr83 signalling mechanisms or other unidentified interactions could have an important physiological role in the control of energy metabolism, particularly after HFD exposure. Furthermore, the observation that Gpr83 ko mice are lean, resistant to diet-induced obesity and -protected from diet-induced glucose intolerance upon HFD exposure supports a role of Gpr83 in the regulation of systemic metabolism that is beyond the modulation of ghrelin action. Collectively, our data identify Gpr83 as a novel, central regulator of ghrelin receptor activity and suggest that in addition to regulating ghrelin signalling, Gpr83 has an important role in the regulation of systemic energy metabolism. Further analyses are required to elucidate the different mechanisms through which Gpr83 exerts these effects, including the specific nature of the molecular interaction with Ghsr1a and other receptors. Generation of receptor constructs Constructs were amplified and cloned into the pcDps vector. Haemagglutinin tags were cloned either at the amino terminus (N-HA) or behind the signal peptide sequence. FLAG-tags were generated at the carboxy terminus (C-FLAG). The pcDps (NHA-rM3R) was kindly provided by Torsten Schöneberg (University of Leipzig), the pcDNA3 (MCFD2-YFP1 and -YFP2) constructs were provided by Hans-Peter Hauri (University of Basel) [13] . MC3R was amplified from human genomic DNA and the GHSR from human complementary DNA (UMR cDNA Resource Center) [14] , [15] . Receptor-YFP1 and -YFP2 fusion genes were generated by replacement of the MCFD2 gene. The pGL4.30 (luc2P/NFAT-RE/Hygro) vector was purchased from Promega. Measurement of inositol-3 phosphate Intracellular inositol-3 phosphate was determined using a luciferase reporter assay (Promega). Receptor DNA (pcDps) and a reporter construct containing a response element and the firefly luciferase gene under control of the nuclear factor of activated T cells were cotransfected and cells were stimulated 2 days after transfection for 6 h at 37 °C with human n -octanoyl ghrelin (C8, AnaSpec), rat (des-octanoyl)-ghrelin (PolyPeptide Laboratories) or rodent obestatin (PolyPeptide Laboratories), and lysed with 100 μl 1 × Passive Lysis Buffer (Promega). Inositol-3 phosphate accumulation was determined by luciferase activity according to the manufacturer’s instructions. Receptor dimerization studies Receptor dimerization was measured using two independent approaches. For sandwich ELISA, HA- and FLAG-tagged constructs were cotransfected in COS-7 and N41 cells. For YFP-PCA, receptor-YFP1 and -YFP2 constructs were cotransfected in HEK293 cells. Cotransfection of MC3R and GHSR was used as positive control, whereas the respective cotransfection with the rM3R was used as a negative control. Cells were collected and solubilized at 4 °C (10 mM Tris/HCl, pH 7.4, 150 mM NaCl, 1 mM EDTA, 1 mM dithiothreitol, 1% deoxycholate-Na, 1% NP-40 and 0.2 mM phenylmethylsulphonyl fluoride) overnight. Lysates were incubated in anti-FLAG antibody-coated 96-well plates for 2 h. The HA epitope was probed with a biotin-labelled antibody. Bound biotin anti-HA antibody was detected using peroxidase-labelled streptavidin (BioLegend) in a substrate/chromogen reaction as described elsewhere [16] . Total protein concentration of lysates was measured using a bicinchoninic acid-based protein assay (Thermo Scientific). Interaction between receptor-YFP1 and -YFP2 constructs reconstitutes the active YFP. A variant of YFP (Q69M) that is characterized by strong photostablility [13] was used. Following collection of the cells, fluorescence was assessed using flow cytometry. Cell surface and total expression studies HA-tagged receptors were transfected into COS-7 cells using 48-well plates (3.75 × 10 4 cells per well). Cells were washed 3 days after transfection, paraformaldehyde-fixed and probed with a biotin-labelled anti-HA antibody (Roche). Bound biotin anti-HA antibody was detected as described [12] . Total receptor expression was measured via sandwich ELISA as described above, using HA- (N-terminal or behind signal peptide sequence) and C-FLAG double-tagged constructs. Generation of global Gpr83 ko mice Gpr83 ko mice were generated as described elsewhere [17] . Briefly, a 2,374kb genomic region containing exons 2 and 3 of the Gpr83 isoform 1 (NM_010287) was deleted by mating Gpr83 floxed mice with mice expressing the cre recombinase under the control of the promine 1 promoter. Genotyping was performed by PCR analysis. Primer 1: 5′-TGGAAATGCCACCCCAGAGC-3′; primer 2: 5′-AGACGGAGATGGGAGCATGC-3′; and primer 3: 5′-TGTGAGCACACACTCCCTGG-3′. Genotyping was confirmed by quantitative PCR analysis by using primers amplifying a coding 175-bp fragment in exons 2/3, which is excised in the ko mice ( Supplementary Fig. S3 ). Ghrelin treatment of Gpr83 ko mice Mice were housed at an ambient temperature of 23 °C with constant humidity and a 12-h light–dark cycle. Mice had free access to water and were, if not indicated otherwise, fed ad libitum with either a regular chow diet (Teklad LM-485) or a HFD (58% kcal fat; Research Diets Inc., New Brunswick, USA). All procedures were approved by the Institutional Animal Care and Use Committee of the University of Cincinnati. Measurements of energy expenditure were performed using a customized indirect calorimetric system (TSE Systems Gmbh, Bad Homburg, Germany). After adaptation for 24 h, recordings were collected over the following 100 h. Body fat and lean tissue mass was assessed using the EchoMRI (Houston, TX, USA). Acute food intake was measured in 12-week-old, chow-fed, male Gpr83 ko ( N =14) and wt ( N =10) mice, and were treated with a single intraperitoneal injection of either rat ghrelin (4.8 μmol kg −1 ) or saline followed by measurement of food intake at 0, 0.5, 1, 2, 4, 8 and 24 h post injection. Ghrelin-induced GH secretion was assessed in 9-week-old chow-fed Gpr83 ko ( N =8) and wt control mice ( N =17). For analysis of GH, mice were injected with a single intraperitoneal injection of rat ghrelin (4.8 μmol kg −1 ) followed by blood sampling at time points 0, 10 and 20 min post injection. Plasma GH levels were assessed using a commercially available ELISA (Millipore, Billerica, MA, USA). Effects of peripheral ghrelin treatment were assessed in 24-week-old, and HFD-fed male Gpr83 ko ( N =16) and wt ( N =8) mice were treated twice daily for 6 consecutive days via subcutaneous injection of either rat ghrelin (2.4 μmol kg −1 per day) or saline. Central effects of ghrelin were assessed in 14-week-old, chow-fed, male Gpr83 ko ( N =14) and wt ( N =12) mice. For icv infusion, rat ghrelin was dissolved in saline and infused at a dose of 5 nmolper day per mouse using osmotic minipumps (1007D; Alzet, Cupertino, CA). For icv surgery, mice were anaesthetized using 5% isoflurane and maintained on 2.5% isoflurane throughout the surgery. Mice were stereotaxically implanted (David Kopf Instruments, Tujunga, CA) with a cannula (Brain Infusion Kit No. 3; Alzet) placed in the lateral cerebral ventricle using the coordinates −0.7 mm posterior to bregma, −1.2 mm lateral to the midsagittal suture and to a depth of −2.5 mm from the surface of the brain, with bregma and lambda being horizontal. A polyethylene catheter attaching the cannula to the minipump was subcutaneously implanted in the interscapular region. The infusion rate of the pumps was 0.5 μl h −1 for 7 days. Directly after surgery, the animals received a single subcutaneous injection of 0.28 mg kg −1 buprenorphine (Buprenex; Reckitt Benckiser Healthcare, Richmond, VA). Assessment of body weight and food intake started the day after the surgery. Body composition (fat and lean tissue mass) was assessed immediately before surgery and after 7 days. Colocalization of Gpr83 with Ghsr and AgRP To check whether Gpr83 is located in neurons expressing Ghsr or AgRP, in situ hybridization histochemistry was performed to visualize the gene expression of Gpr83; immunohistochemistry of β-galactosidase, the products of lacZ gene driven by the Ghsr promoter in Ghsr ko mice [18] , was used to visualize the Ghsr. Immunohistochemistry of AgRP neurons were performed in fasted mouse ARC. Ghsr ko mice or 16-h fasted wt mice were perfused transcardially with diethylpyrocarbonate-treated 0.9% NaCl followed by 4% 4 °C paraformaldehyde. After post-fixation and saturation with 30% sucrose, brains were cut by cryostat into 25 μm. Sections were treated by 0.1 M PBS-buffered methanol and H 2 O 2 for 10 min, 0.2 N HCl for 10 min, 0.2% glycine buffer 30 s and 0.1% Triton X-100 for 10 min. Brain sections were hybridized in hybridization buffer (Sigma-Aldrich, USA) containing 100 nM locked nucleic acid (LNA) – modified cDNA probes labelled with digoxigenin (5′-AGAGAGAAGAAGGTAGCCATGA-3′) (Exiqon, Denmark) in 52 °C for 8 h. After stringent washing in SSC buffer in 52 °C and final washing in 0.1 M PBS, sections were then coincubated with sheep anti-digoxigenin antibody (1:200, Abcam, USA) and chicken anti-β-galactosidase (1:200, Abcam) or goat-anti AgRP antibody (R&D) in 4 °C over night. Sections were incubated with biotinylated anti-sheep secondary antibody for an hour and then incubated with either streptavidin conjugated with DyLight 488 (1:200, for Gpr83) and donkey anti-chicken antibody conjugated by Cy3 (1:300, for β-galactosidase), or incubated with streptavidin-conjugated Cy3 (1:200, for Gpr83) and horse anti-goat antibody conjugated by DyLight 488 (1:300, for AgRP) (all from Jackson ImmunoResearch Laboratories, USA). After thorough rinsing, sections were mounted with mounting medium and visualized by confocal microscopy. Analysis of plasma samples Plasma total immunoreactive insulin and leptin were measured with Multiplex Luminex xMAP assay (Millipore Corporation, Massachusetts, USA). The lower and upper limits of detection were 68.5 and 50,000 pg ml −1 , with minimum detectable concentrations of 25 and 22 pg ml −1 . Plasma triglycerides and total cholesterol were determined using commercially available kits from ThermoFisher Scientific Inc. (Virginia, USA). Plasma FFA levels were determined using kits from Wako Chemical Inc. (Richmond, Virginia, USA), according to the manufacturer’s instructions. Total IGF-I (mouse high-sensitivity IGF-I; IDS, Boldon, UK) and GH (Mediagnost, Reutlingen, Germany) were analysed in plasma samples using commercially available immunoassays, according to the manufacturer’s instructions. Plasma levels of desacyl and acyl ghrelin were assessed in 28-week-old Gpr83 ko ( N =16) and wt mice ( N =7) fed with an HFD diet for 15 weeks as described previously [19] . Data analysis Analyses were performed using Graph Pad Prism (GraphPad Software, San Diego, California, USA). Differences between treatment groups were assessed by two-way analysis of variance followed by Dunnett’s or Bonferroni’s post hoc test, one-way analysis of variancefollowed by Bonferroni’s or Newman Keuls’ post-hoc test, or unpaired two-tailed Student’s t -test. Data for energy expenditure were analysed using analysis of covariance by using body mass as a covariate. All results are given as means±s.e.m. Results were considered statistically significant when P <0.05, with the significance level indicated as * P <0.05, ** P <0.01 and *** P <0.001. How to cite this article: Müller, T. D. et al. The orphan receptor Gpr83 regulates systemic energy metabolism via ghrelin-dependent and ghrelin-independent mechanisms. Nat. Commun . 4:1968 doi: 10.1038/ncomms2968 (2013).